Three-dimensional imaging of magnetic domains Magnetic domains have been the subject of much scientific investigation since their theoretical existence was first postulated by P.-E. Weiss over a century ago. Up to now, the three-dimensional (3D) domain structure of bulk magnets has never been observed owing to the lack of appropriate experimental methods. Domain analysis in bulk matter thus remains one of the most challenging tasks in research on magnetic materials. All current domain observation methods are limited to studying surface domains or thin magnetic films. As the properties of magnetic materials are strongly affected by their domain structure, the development of a technique capable of investigating the shape, size and distribution of individual domains in three dimensions is of great importance. Here, we show that the novel technique of Talbot-Lau neutron tomography with inverted geometry enables direct imaging of the 3D network of magnetic domains within the bulk of FeSi crystals. Magnetic domains and their substructures link fundamental physical properties (for example, anisotropy) with the macroscopic properties (for example, magnetization) [1] , [2] . A complete understanding of macroscopic effects, such as noise and energy loss characteristics in magnetic devices, is almost impossible without knowledge of the underlying domain structure [2] . This necessity for domain analysis has hastened the improvement of classical domain observation techniques such as the Bitter method, magneto-optical Kerr microscopy and various methods based on electron microscopy, and has also led to the development of new methods such as magnetic force microscopy, spin-polarized tunnelling microscopy and X-ray spectroscopic techniques [2] , [3] , [4] . However, all these methods are intrinsically limited to two-dimensional (2D) imaging of either thin films (transmission techniques) or the surface domains of thick specimens (reflection techniques); access to the volume domains in the bulk of opaque (metallic) magnetic materials is not possible. However, in most applications, such as transformers, electro-motors and other inductive devices, it is the (basic) volume domains that are responsible for key magnetic properties (for example, susceptibility and energy loss). 3D analysis of the volume domains in bulk materials is therefore an important step towards understanding fundamental magnetic properties and developing and improving materials in a targeted manner. Simply slicing a sample to investigate the interior domains is meaningless, as a new domain pattern related to the new surface will form immediately. The only exception, though with very little impact on the volume domain information gained, is a destructive technique introduced by Libovický, which, however, only works for a special FeSi alloy at elevated temperatures [5] . Owing to the lack of experimental techniques, our understanding of volume domains has so far been based on a combination of surface observation and domain theory. This combined analysis works reasonably well for bulk samples with ideally orientated or slightly misoriented surfaces (meaning that the easy axes of magnetization are either parallel to the surface or off by only a few degrees). In the general case of arbitrarily oriented surfaces, complex surface domains are formed that give no hint of the volume domains hidden beneath. Numerical micromagnetic calculations, though increasingly and very successfully applied to small particles and film elements, are unsuitable for domain analyses in bulk materials. X-ray topography allows investigation of the interior of bulk samples without cutting, but is limited to thin crystals and reveals little additional information [6] . Neutrons on the other hand have a long and outstanding history of probing magnetic phenomena in bulk samples. As charge-free particles, they are able to penetrate thick layers of metals although being sensitive to magnetic fields due to their intrinsic magnetic moment. However, current techniques have severe limitations; (2D) polarized neutron topography is very limited in contrast and spatial resolutions, while polarized neutron imaging—based on the measurement of spin precession angles—is limited to weak magnetic fields ( ∼ 1 mT) in the case of bulk samples [7] , [8] . In the late 1990s, Podurets et al . [9] used a double crystal diffractometer to demonstrate that domain walls oriented almost parallel to the neutron beam direction can be visualized, but this proved very time consuming. Well-aligned domain walls in a thin ferromagnetic plate have also been investigated using the superior method of phase grating interferometry for (2D) neutron dark-field imaging [10] , [11] , [12] , [13] . In both cases, the image contrast is based on the refraction of neutrons at domain walls [14] . Magnetic fields with a flux density B add to the interaction potential of a magnetic medium and hence contribute to the refractive index with the spin-dependent term δ μ =± μB/ 2 E 0 =±2 μBmλ 2 /h 2 , where μ is the magnetic moment, E 0 the unperturbed kinetic energy, λ the neutron wavelength, m the mass of the neutron and h the Planck's constant. The different Zeeman energies ± μB cause corresponding deviations in the momentum transfer for parallel and anti-parallel spin orientations with respect to the magnetic flux density B. The spin states therefore split by refraction when a neutron beam passes a domain wall that can be considered thin, that is, ω ≥ ω L , where ω equals the effective rotation frequency corresponding to the field B a neutron experiences if it passes the Bloch wall, and ω L is the Larmor frequency of the neutron [14] , [15] . Because this field-dependent refraction is in the ultra-small angle range (for typical neutron wavelengths around a few Å), it can only be detected using high angular resolutions and grazing incidence of the beam to the Bloch wall [15] , [16] . Consequently, only domain walls nearly parallel to the beam, and therefore only a very limited number of such walls are detected by these (2D) measurements. Here, we apply a tomographic approach based on a modified Talbot-Lau neutron imaging set-up with inverted geometry. This method makes it possible to map the full entity of domain walls in the bulk of massive samples and thus reveals the domain structure beyond the surface region non-destructively. Owing to the high penetration depth of neutrons, this not only expands potential investigations to the third dimension, but also increases the accessible depth to several centimetres for ferromagnetic materials such as iron or steel. In particular, we visualize and analyse quantitatively the 3D shape and distribution of individual domains in a misoriented magnetic FeSi crystal. We find a square-root dependence of the volume domain width on the sample thickness, which agrees with current theoretical predictions. Imaging magnetic domain walls For our investigation, we chose Fe 12.8-at%Si single crystals ( Fig. 1a ). This alloy is characterized by a low (negative) magnetostriction constant and a crystal anisotropy that is about 1.5×10 4 J m −3 (pure iron=4.6×10 4 J m −3 ). In terms of the domain properties, this material can be considered 'iron-like', that is, the (100) directions are the easy axes of magnetization. One of our goals was to investigate the dependence of the bulk domain width on the crystal thickness. As the surface domains are highly complex in such misorientations (see Methods section), the bulk domain width cannot be inferred from surface observations for crystal thicknesses beyond several 100 μm. 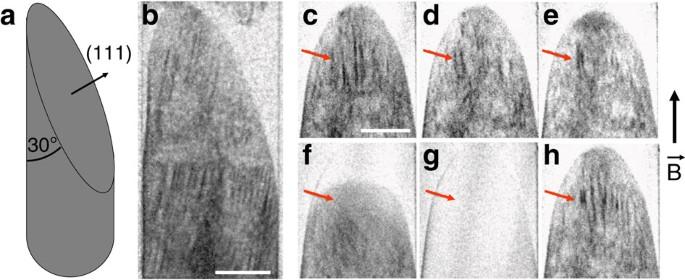Figure 1: Talbot-Lau neutron radiographies of magnetic domains. (a) Sketch of the investigated FeSi wedge (a). (b) Radiographic projection images of the wedge as obtained by Talbot-Lau neutron dark-field radiography. The dark stripes are caused by domain walls that are aligned almost parallel to the incident beam. Scale bar: 3 mm. The wedge was placed in an external magnetic field (parallel to the cylinder axis) of 11 mT (c), 20 mT (d), 40 mT (e), 84 mT (f), 225 mT (g) and 11 mT (h). Scale bar (c–h): 3 mm. With increasing field strength, a movement can be observed in the domain walls (red arrows). At 84 mT (f), most large domains are aligned along the magnetic field lines. The remaining dark background is caused by small surface and (branched) subsurface domains, which are saturated at 225 mT (g). When the magnetic field strength is returned to the initial value, a domain wall configuration very similar to the initial one can be observed (h). Figure 1: Talbot-Lau neutron radiographies of magnetic domains. ( a ) Sketch of the investigated FeSi wedge ( a ). ( b ) Radiographic projection images of the wedge as obtained by Talbot-Lau neutron dark-field radiography. The dark stripes are caused by domain walls that are aligned almost parallel to the incident beam. Scale bar: 3 mm. The wedge was placed in an external magnetic field (parallel to the cylinder axis) of 11 mT ( c ), 20 mT ( d ), 40 mT ( e ), 84 mT ( f ), 225 mT ( g ) and 11 mT ( h ). Scale bar ( c – h ): 3 mm. With increasing field strength, a movement can be observed in the domain walls (red arrows). At 84 mT ( f ), most large domains are aligned along the magnetic field lines. The remaining dark background is caused by small surface and (branched) subsurface domains, which are saturated at 225 mT ( g ). When the magnetic field strength is returned to the initial value, a domain wall configuration very similar to the initial one can be observed ( h ). Full size image A typical radiographic projection of one of the FeSi wedges as obtained by our method is shown in Figure 1b (a detailed explanation of the method is given in the Methods section and in Supplementary Fig. S1 ). Following the argument outlined above, the dark stripes should be assignable to scattering at individual domain walls. To prove this, the FeSi sample was exposed to magnetic fields. With increasing magnetic field strength, the domain structure can be seen to change and the domain walls move ( Fig. 1c–e ). At around 84±5 mT, the central part of the crystal is magnetically almost saturated, which is expressed by the disappearance of visible domain walls ( Fig. 1f ). By increasing the field strength yet further, the diffuse signal, which can be assigned to the small remaining surface and (branched) subsurface domains, begins to vanish because of ongoing saturation of the surface regions ( Fig. 1g ). After decreasing the magnetic field strength to the initial value, the domains rearrange themselves into a structure closely resembling the initial one ( Fig. 1h ). 3D imaging In contrast to radiography, tomographic reconstruction reveals the full set of domain walls in the sample accessible within the spatial resolution (about 35 μm). 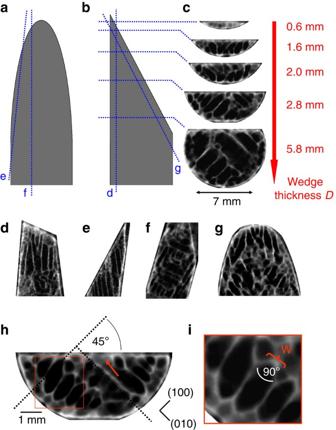Figure 2: Talbot-Lau neutron tomography of a FeSi wedge. (a,b) Sketches of the FeSi wedge (a, front view andb, side view). (c) Horizontal slices at different wedge thicknesses as indicated inb. (d–g) Cross-sections through the Talbot-Lau neutron tomogram along different planes (dotted by d–g inaandb) that show the high complexity of the 3D shape of magnetic domains. (h) Horizontal slice (as inc). (i) Enlargement of the area marked in red inh. Small domains that cannot be spatially resolved lead to a more or less homogenous dark-field signal (light grey areas, see red arrow inhas an example) where no individual domain walls can be identified clearly. A similar effect occurs whenever a domain wall that is blurred by the limited spatial resolution lies in the plane of the slice. The images in Figure 2 show several cross-sections through the volumetric data set perpendicular to the cylinder axis taken at different wedge widths ( Fig. 2c ) and along some additional planes ( Fig. 2d–i ). Typical domain shapes can be identified, and domain widths W of up to 1 mm are found. Figure 2: Talbot-Lau neutron tomography of a FeSi wedge. ( a , b ) Sketches of the FeSi wedge ( a , front view and b , side view). ( c ) Horizontal slices at different wedge thicknesses as indicated in b . ( d – g ) Cross-sections through the Talbot-Lau neutron tomogram along different planes (dotted by d–g in a and b ) that show the high complexity of the 3D shape of magnetic domains. ( h ) Horizontal slice (as in c ). ( i ) Enlargement of the area marked in red in h . Small domains that cannot be spatially resolved lead to a more or less homogenous dark-field signal (light grey areas, see red arrow in h as an example) where no individual domain walls can be identified clearly. A similar effect occurs whenever a domain wall that is blurred by the limited spatial resolution lies in the plane of the slice. Full size image However, the different cross-sections in Figure 2 also reveal how the geometries differ depending on the plane and angle of the cross-section. This becomes most obvious when representing a selected number of domains three-dimensionally and extracting the volume of single domains. 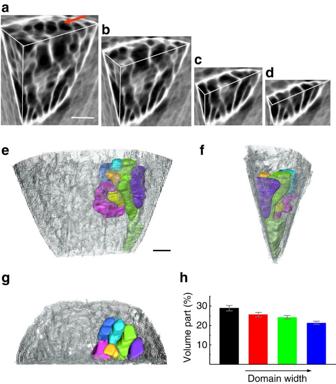Figure 3: 3D analysis of individual domain shapes. (a) 3D view on the sliced tomography of the FeSi wedge. The tomographic representation of the wedge (not the wedge itself) was cut along thex–y,y–zandx–zplanes. (b–d) The tomogram is cut stepwise from the top. Scale bar (a–d): 1 mm. (e–g) Some individual domains (marked by a red arrow ina) were extracted from the 3D volume and are displayed in different (arbitrary) colours. The surface of the wedge is shown in semi-transparent grey. Scale bar (e–g): 1 mm. (h) An analysis of the domain volume reveals that the majority of the entire volume consists of comparably large domains with a width of more than 300 μm. The four columns represent the volume parts of domains with widths of the <300 μm (black column), 300–600 μm (red column), 600–900 μm (green column) and >900 μm (blue column). Figure 3a–d shows 3D views of the inner structure of the wedge, and Figure 3e–g shows the shape and arrangement of several extracted domains within the wedge. Figure 3: 3D analysis of individual domain shapes. ( a ) 3D view on the sliced tomography of the FeSi wedge. The tomographic representation of the wedge (not the wedge itself) was cut along the x – y , y – z and x – z planes. ( b – d ) The tomogram is cut stepwise from the top. Scale bar ( a – d ): 1 mm. ( e – g ) Some individual domains (marked by a red arrow in a ) were extracted from the 3D volume and are displayed in different (arbitrary) colours. The surface of the wedge is shown in semi-transparent grey. Scale bar ( e – g ): 1 mm. ( h ) An analysis of the domain volume reveals that the majority of the entire volume consists of comparably large domains with a width of more than 300 μm. The four columns represent the volume parts of domains with widths of the <300 μm (black column), 300–600 μm (red column), 600–900 μm (green column) and >900 μm (blue column). Full size image From the domain shape and wall arrangement, 90 and 180° walls can be separated in many cases. For example, Figure 2h,i clearly shows a preferred orientation of the domain walls. Most walls are orientated along angles around 45 and 135° (with respect to the sample's reference system). It can be concluded that these are 180° domain walls (that is, with anti-parallel magnetization directions in adjacent domains) that are oriented parallel to the (100) crystallographic directions [2] . The extracted domains were used for further quantitative analysis of the domain size distribution ( Fig. 3h ). Most of the volume of the wedge consists of large domains with widths of several 100 μm and typical volumes ranging from 0.03 mm 3 to more than 1 mm 3 . The entire sample volume is filled by domains with widths of <300, 300–600, 600–900 and >900 μm in approximately equal fractions. 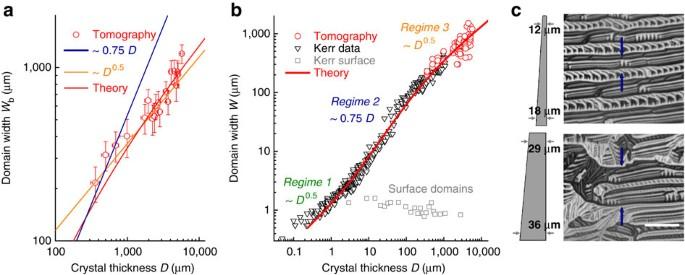Figure 4: Dependence of the volume domain width on the sample thickness. (a) Widths of the magnetic domains at different sample thicknesses as obtained from the tomographic data set (mean values). (b) Combined Kerr microscopic and tomographic data for the domain width dependence on crystal thickness in FeSi. The data show three different regimes. A fit based on equation (1) is given inaandb. (c) Kerr image of surface domains showing the fine closure domains of an underlying fractal domain pattern that is coarsened in an iterative way towards the volume (Supplementary Fig. S2). The depth of the branched domains extends to about 50 μm away from the surface2. The volume domains yield a superstructure in the surface domain pattern, which can be used to extract the volume domain width up to a crystal thickness of several 100 μm. This is demonstrated for sample thicknesses of 12–18 μm (top) and 29–36 μm (bottom). Black numbers give the local wedge thickness perpendicular to the plane of view, indicated by the grey arrows. The spacing between the blue arrows represents domain width, and it is 9 μm in the top panel and 23 μm in the bottom panel. The Scale bar represents a length of 20 μm. Domain size analysis The tomographic cross-sections in Figure 2c reveal a clear trend towards increasing domain sizes at larger wedge thickness, which becomes even clearer in the detailed analysis presented in Figure 4a . Indeed, a strong correlation is to be expected between the domain width W and the thickness D of the sample [2] . Domain theory predicts three regimes for the dependence of domain width on crystal thickness in iron-like materials. (i) Up to a thickness of several μm, W ∼ √ D (regime 1). (ii) Beyond this thickness, the phenomenon of domain branching sets in. The domains are refined towards the crystal surface in an iterative way to avoid magnetic poles at the surface and to reduce the volume of the outermost (unfavourably magnetized) closure domains, while at the same time saving wall energy in the volume. The volume domain width scales with W ∼ D over several orders of crystal thickness (regime 2). (iii) For very large thicknesses a W ∼ √ D behaviour is expected again (regime 3), which is dominated by the magnetostrictive self energy of the branched subsurface domains (1). A detailed explanation is given in the Supplementary Methods and in Supplementary Figure S2 . Figure 4: Dependence of the volume domain width on the sample thickness. ( a ) Widths of the magnetic domains at different sample thicknesses as obtained from the tomographic data set (mean values). ( b ) Combined Kerr microscopic and tomographic data for the domain width dependence on crystal thickness in FeSi. The data show three different regimes. A fit based on equation (1) is given in a and b . ( c ) Kerr image of surface domains showing the fine closure domains of an underlying fractal domain pattern that is coarsened in an iterative way towards the volume ( Supplementary Fig. S2 ). The depth of the branched domains extends to about 50 μm away from the surface [2] . The volume domains yield a superstructure in the surface domain pattern, which can be used to extract the volume domain width up to a crystal thickness of several 100 μm. This is demonstrated for sample thicknesses of 12–18 μm (top) and 29–36 μm (bottom). Black numbers give the local wedge thickness perpendicular to the plane of view, indicated by the grey arrows. The spacing between the blue arrows represents domain width, and it is 9 μm in the top panel and 23 μm in the bottom panel. The Scale bar represents a length of 20 μm. Full size image The correlation between the bulk domain width W b and D can be described by the following equation [2] : where C p is the 'quasi-closure' coefficient, γ w the specific wall energy, C s a geometry-dependent factor and G m describes the maximum rate (speed) of the domain width that is rising from its surface width W s to its bulk value W b ( Supplementary Methods and Supplementary Fig. S2 ). In the investigated FeSi crystal, the three expected regimes of thickness dependence can be observed ( Fig. 4b ) by combining results obtained by Kerr microscopy with the data measured by Talbot-Lau neutron tomography. A fit of our experimental data with the function given in equation (1) yields: G m =1.5, C s =933 and C p =3 J m −3 . (The specific wall energy of the 180° basic domain walls was assumed to be γ w =1.3×10 −2 J m −3 , calculated from γ w =2 √( AK c ), with the exchange constant A =2.1×10 −11 J m −1 and the first-order anisotropy constant K c =2×10 4 J m −3 .) The domain width data ( Fig. 4a,b ) obtained by Talbot-Lau neutron tomography clearly support a W ∼ √ D dependence in regime 3, which is not accessible by Kerr microscopy because of its restriction to surface domains. This is the first experimental proof for the theoretical predictions. For small crystal thicknesses, the volume domains can be seen indirectly as a 'superstructure' in the otherwise strongly branched surface patterns of a Kerr microscopic image ( Fig. 4c ). In this way, the widths of these volume domains can be estimated up to wedge thicknesses of several 100 μm ( Fig. 4b ). In the region where the data points overlap, Kerr measurement and Talbot-Lau neutron tomography results are in good agreement. This proves the reliability of this novel 3D neutron imaging method and demonstrates its potential for providing width analyses based on real 3D data sets and for extending the accessible sample thickness range. By introducing Talbot-Lau neutron tomography with inverted geometry, we have opened the door to true 3D imaging of magnetic domains, which is not feasible using any other technique. Such tomography extends and complements the capabilities of conventional methods that are limited to the 2D imaging of domains in magnetic films and on surfaces. The possibility to study the 3D anatomy of magnetic microstructures paves the way to future applications in various fields, as domains and magnetization processes can now be studied even if they are hidden by surface coatings or by complex surface domain patterns. The flexibility of the experimental setup permits an easy sample manipulation, for example, by magnetic fields, mechanical stresses or temperatures. It is further expected that the method can be applied to the imaging of magnetic phase transitions, magnetic or superconducting froths, superconductive ferromagnets and flux-pinning/-trapping in superconductors. As a first example for the successful application of the method, we have presented an analysis of the 3D domain structure in a FeSi crystal and could establish the correlation between domain size and sample thickness over six orders of magnitude by combined tomography and Kerr microscopy. We investigated a hitherto experimentally unexplored regime in which the domain size scales as the square root of sample thickness, thus confirming the theoretical prediction that the domain-branching mechanism is altered at volume domain sizes larger than several 100 μm. Domain growth returns to the square root dependence known for domain sizes below 1 μm. This indicates that for large crystal thickness, the iterative addition of new domain generations in the surface region is stopped. As significant increases in spatial resolution (imaging detectors with pixel sizes as small as 2.5 μm) have been reported [17] , and available neutron flux density (achievable through advances in neutron optics [18] for imaging) are expected in the near future, even branched domains close to the surface will become observable with this 3D imaging technique. The technique might also be combined with other imaging methods such as electron microscopy [19] or (soft) X-ray tomography. Experimental set-up The measurements were carried out with a grating-based shearing interferometer based on the principle of Talbot-Lau interferometry [20] , [21] . The set-up used is shown schematically in Supplementary Figure S1a . It consists of three gratings [10] , [12] . (i) The source grating, G S , is an array of slits within an absorbing gadolinium mask with a period, p S , of 790 μm. This grid produces several individually coherent beams. (ii) The phase grating, G Ph , is (almost) transparent and has a much smaller period, p Ph , of 7.96 μm. It causes a phase shift of λ /2 between the incoming adjacent rays and produces a diffraction pattern with a period of about p Ph /2 in the first fractional Talbot distance. (iii) The analyser grating, G A , is an absorption grating similar to G S , but with a period of 4 μm (about p Ph /2). This grating is used to detect the interference pattern, which is much smaller than the detector resolution (pixel size). This grating (or, alternatively, grating G S ) is scanned horizontally in steps parallel to the phase grating to measure the entire pattern across each image pixel. The amplitude damping of the measured transmission function is the so-called dark-field signal ( Supplementary Fig. S1b ), the intensity of which is increased by refraction at magnetic domain walls present in any sample placed between G S and G A . By stepwise rotation (360°) of the sample around the vertical axis, several projection images are taken [13] that contain information about all magnetic domain walls in the sample (limited only by the spatial resolution). The gratings have an area size of ∼ 64×64 mm 2 (details about the fabrication process are given in ref. 22 ). The distance between gratings G S and G Ph was 4,500 mm, and that between gratings G Ph and G A was 22.7 mm (that is, the first fractional Talbot distance for a wavelength of 3.5 Å). The set-up was combined with a state-of-the-art high-resolution neutron tomography detector system (V7-CONRAD instrument at the Helmholtz Centre Berlin for Materials and Energy) [23] providing a spatial resolution of 35 μm (pixel size 13.5 μm). In all, 100 image sets were recorded at 100 equidistant angles over a range of 360°. Each image set contained 14 radiographs corresponding to different positions of the analyser grating. An exposure time of 100 s per radiographic image was chosen. The data set was corrected by additional background and flat field measurements, and the dark-field signal was evaluated by a sinusoidal fitting routine [13] , [10] . Talbot-Lau neutron tomography with inverted geometry In contrast to recently introduced imaging methods based on the Talbot-Lau technique [10] , [11] , significant modifications were necessary to enable imaging of magnetic domains in the bulk and in three dimensions. In particular, the extinction of the analysed interference pattern caused by the signal accumulation because of a great number of domain walls at the surface and in the bulk, as well as limitations in the spatial resolution and signal intensity had to be addressed ( Supplementary Fig. S1c ). For these reasons, we altered the geometry of the standard Talbot-Lau set-up and inverted the locations of the sample and the phase grating. In conventional Talbot-Lau set-ups, the sample is placed in the approximated plane wave field of the partially coherent beams originating from the source grating, that is, between source grating and phase grating (see red arrow in Supplementary Fig. S1 ). In the novel approach of the inverted geometry, the sample is placed directly into the interfering wave field between the phase and analyser gratings ( Supplementary Fig. S1a ). This inverted geometry reduces the dark-field contrast and prevents contrast saturation. Image contrast can be adjusted by varying the sample-to-analyser (grating) distance. Furthermore, the spatial resolution is significantly increased because neutron spot blurring on the detector—caused by beam divergence—is decreased by reducing the sample-detector separation. This also allows larger pinholes to be used for the incoming beam (while maintaining high spatial resolution) and thus leads to higher beam intensities (shorter exposure times). The second significant modification of the set-up was the application of a broad cold neutron spectrum (referred to as 'white beam') instead of a (quasi-) monochromatic beam, where the selected wavelength matches the interference condition for the first fractional Talbot distance. This has two major advantages: (i) the available beam intensity is significantly increased (by about one order of magnitude), which is especially important for high-resolution tomography measurements and (ii) although the original contrast of the interference pattern at the first fractional Talbot distance is reduced, the strongly wavelength-dependent dark-field signal remains highly sensitive (because of long wavelength contributions), although dark-field contrast saturation is prevented (because of short wavelength partitions). To underline this, two images taken with the new and a standard set-up are shown in Supplementary Figure S1c,d , respectively. Tomographic data reconstruction For a successful 3D reconstruction of the domain structure, a dedicated algorithm had to be developed. Although image contrast is achieved through dark-field evaluation, it originates from refraction and thus involves a significant angular dependence (comparable to (synchrotron) X-ray phase contrast tomography with edge enhancement) [13] , [15] , [24] , [25] . However, we applied our own iterative reconstruction algorithm (DIRECTT), which is especially suitable for incomplete data sets such as missing projection angles and insufficient transmission intensities [26] . It is essential to dampen the strong signals produced by a structure at specific angles to avoid image artefacts [24] . 3D rendering of the reconstructed cross-sectional slices was completed using the commercial software packages AVIZO and VGStudioMax. FeSi samples Cylindrical rods (Fe 12.8-at%Si single crystals) with 7-mm diameter and 15–20-mm length were grown by zone melting. From such rods, a wedge-shaped sample was cut with an electro-erosive saw. The wedge had an inclination angle of 30° ( Fig. 1a ), with its thickness increasing from 0 to 7 mm over a distance of ≈14 mm. One principal surface (the inclined) was in the (111)-orientation, which is an extremely misoriented surface for iron-like materials. How to cite this article: Manke, I. et al . Three-dimensional imaging of magnetic domains. Nat. Commun. 1:125 doi: 10.1038/ncomms1125 (2010).